The COG1-OsSERL2 complex senses cold to trigger signaling network for chilling tolerance injaponicarice 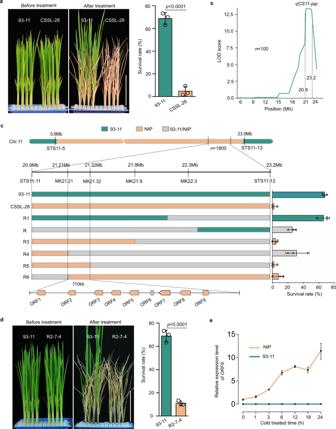Fig. 1: Map-based cloning of the major gene inqCS11-jap. aChilling tolerance of 93-11 (indica) and of chromosome segment substitution line 28 (CSSL-28). The survival rates were determined after a 4-week recovery period. Data are means ± SD (two-tailed Student’st-test;n= 3 biological replicates). Scale bars = 6 cm.bLocation ofqCS11-japon chromosome 11 revealing by LOD score plots.cFine mapping of theqCS11-japlocus. Left, high resolution mapping. STS11-5, STS11-11, MK21.21, MK21.32, MK21.9, MK22.3, STS11-12 and STS11-13 were molecular markers (Supplementary Data5). Right, survival rates of six recombinants (R1–R6) and the parents. Data are means ± SD (n = 3 biological replicates).dChilling tolerance of 93-11 and a homozygous recombinant line (R2-7-4). Data are means ± SD (two-tailed Student’st-test;n= 3 biological replicates). Scale bars = 6 cm.eThe expression levels ofORF9(LOC_Os11g36200) in 93-11 and Nipponbare (NIP) with different treatment times at 4 °C. Data are means ± SD (n= 3 biological replicates). See also Supplementary Fig.1. Source data are provided as a Source Data file. Improvement of chilling tolerance is a key strategy to face potential menace from abnormal temperature in rice production, which depends on the signaling network triggered by receptors. However, little is known about the QTL genes encoding membrane complexes for sensing cold. Here, C hilling-t o lerance in G engdao / japonica rice 1 ( COG1 ) is isolated from a chromosome segment substitution line containing a QTL ( qCS11-jap ) for chilling sensitivity. The major gene COG1 is found to confer chilling tolerance in japonica rice. In natural rice populations, only the haplogroup1 encodes a functional COG1. Evolutionary analysis show that COG1 originates from Chinese O. Rufipogon and is fixed in japonica rice during domestication. COG1, a membrane-localized LRR-RLP, targets and activates the kinase OsSERL2 in a cold-induced manner, promoting chilling tolerance. Furthermore, the cold signal transmitted by COG1-OsSERL2 activates OsMAPK3 in the cytoplasm. Our findings reveal a cold-sensing complex, which mediates signaling network for the chilling defense in rice. Rice ( Oryza sativa L.) is a major food crop that feeds half of the world’s population. But temperature stress (such as chilling) threatens rice production [1] , [2] ; low temperature is one of the major environmental factors that limits the geographic distribution of rice cultivation [2] , [3] , [4] . And temperature fluctuations have become increasingly intense and frequent caused by the global climate change [5] , [6] . Evolutionarily, cultivated rice originated from wild accessions in the subtropical regions of Asia, and subsequently expanded to a wide latitudinal range [7] . Domesticated rice, including the major subspecies japonica and indica , are characterized by specific climate adaptations based on agro-ecological cultivation conditions [8] . Therefore, molecular genetic tools have been urgently sought to improve chilling tolerance of rice to fight climate change and expand it into northern areas with relatively low yearly temperatures. Chilling tolerance during rice growth and development is a quantitative trait controlled by multiple genetic factors. Delineation of the genetic basis underlying chilling tolerance in rice is still in its infancy. A number of quantitative trait loci (QTLs) that confer chilling tolerance have been mapped, and some major genes have been genetically characterized [2] , [3] , [4] , [9] , [10] . But less is known about the molecular basis underlying the divergence of environmental adaptations and geographical distribution between japonica and indica varieties. Receptors on the plasma membrane recognize exogenous and endogenous signals to trigger appropriate cellular responses during plant growth and development. Leucine-rich repeat receptor like proteins (LRR-RLPs) are a plant membrane protein family, members of which have an extracellular LRR domain but lack an intracellular kinase domain [11] . LRR-RLPs reportedly function in plant development. For example, AtRLP17/TOO MANY MOUTHS, AtRLP10/CLAVATA2, and AtRLP44 participate in stomatal development, maintenance of the apical meristem, and cell wall perturbations, respectively, in Arabidopsis [12] , [13] , [14] . Other members of LRR-RLPs were reported to be involved in Arabidopsis immune response such as AtRLP1, AtRLP23, AtRL30, AtRLP42, and AtRLP51 [15] , [16] , [17] , [18] , [19] . In rice, OsRLP1 associates with its adapter kinase OsSOBIR1 to mediate plant immunity against viral infection [20] . AtLRRop2 is involved in either the chilling or freezing stress response in Arabidopsis [21] . However, it is unknown how such LRR-RLPs sense environmental cold for the tolerance in rice. In the absence of a kinase domain, LRR-RLP likely acts as a receptor or regulator, transmitting signals by forming complexes with somatic embryogenesis receptor kinases (SERKs) and other transmembrane or membrane associated proteins [22] , [23] . SERKs are a subgroup of leucine-rich repeat receptor-like kinases (LRR-RLKs) that operate as co-receptors of various RLKs and RLPs to regulate immunity, growth, and development [23] . In Arabidopsis, AtSERK3/ B RI1- A SSOCIATED RECEPTOR K INASE 1 not only acts as a co-receptor of BRI1 and FLS2, affecting the brassinosteroid and immune signaling pathway, respectively [24] , [25] ; but also acts as a co-receptor of AtRLP17 in stomatal development, of AtRLP44 in cell wall integrity regulation and of AtRLP23 in immune activation [12] , [13] , [14] . In addition, AtSERK3 homologs, namely AtCIKs, act as co-receptors for AtRLP10 [26] . In tomato, S1SERK3 is required for the RLP proteins Cf-9, Cf-2, CF-4, Cf-5, LeEIX1/2, and Ve1 to mediate immune activation [22] , [27] . The rice genome contains two SERK and seven SERK-like ( SERL ) genes that have roles in rice development [28] ( http://rice.uga.edu/ ). However, it is unclear whether SERKs/SERLs form complexes with LRR-RLPs to transmit signals in rice. Cold temperature triggers plasma membrane rigidification, Ca 2+ channel or activation of RLKs/RLPs in plant cells. This signaling subsequently leads to the activation of kinase in the cytoplasm [2] , [29] , [30] . For example, cold stress activates kinase activity of the plasma membrane-localized proteins CRPK1 and CPK28 to promote phosphorylation of 14-3-3 proteins and NLP7, respectively, in the cytosol [31] , [32] . Receptor like kinases CRLK1 and CRLK2 activate the MEKK1-MKK1/2-MPK4 cascade under cold stress to enhance freezing tolerance in Arabidopsis [33] . Similarly, unknown activators in the plasma membrane rapidly activate the MKK4/5-MPK3/6 cascade in response to cold stress, negatively regulating cold tolerance [34] . In rice, the cold-activated OsMAPK3 phosphorylates the transcription factor OsbHLH002 to enhance chilling tolerance [35] . Another cytoplasmic kinase, OsSAPK6, phosphorylates IPA1 to activate chilling tolerance responses [36] . However, the identities of specific plasma membrane activators, such as LRR-RLP/RLK complexes, that activate kinases in the cytoplasm to respond to chilling signals for tolerance in rice are unknown. Here, we characterized C hilling-t o lerance in G engdao/japonica rice 1 ( COG1 ), a major gene identified in a QTL for positive regulation of chilling tolerance in japonica rice. Our data suggested that a functional COG1 allele originated from Chinese populations of O. rufipogon and was under selection during japonica rice domestication. COG1 was determined to be an LRR-RLP and to form a complex with OsSERL2, regulating activation of the latter for sensing cold signals in the membrane. Furthermore, the COG1-OsSERL2 complex activated OsMAPK3 to modulate chilling tolerance. These findings are significant not only in shedding light on the cold signals network but also in the potential for the genetic improvement for the trait in rice breeding. Map-based cloning of QTLs from chromosome segment substitution lines In order to elucidate the genetic basis for rice chilling tolerance divergence, a wide population consisting of 128 chromosome segment substitution lines (CSSLs) was generated by crossing and back-crossing using the chilling-sensitive indica variety 93-11 as the recurrent parent and the chilling-tolerant japonica variety Nipponbare as the donor parent [37] . Then, 72 of 128 individual lines were randomly selected from the CSSLs population to test their cold tolerance. After the seedlings were treated at 4 °C for 44 h, the survival rates of all selected lines ranged from 60–95%, except for CSSL-28, this line had a survival rate of ~5% (Fig. 1a and Supplementary Fig. 1a ). The CSSL-28 was selected for further analysis due to its chilling sensitivity. Molecular markers assay showed that the substituted chromosome segment from Nipponbare was located between 5.6 and 23.9 Mb on chromosome 11 in CSSL-28. These results suggested that the japonica insertion of the CSSL-28 may involve a putative q uantitative trait locus from jap onica rice conferring C hilling S ensitivity on indica rice in chromosome 11 ( qCS11-jap ). Fig. 1: Map-based cloning of the major gene in qCS11-jap . a Chilling tolerance of 93-11 ( indica ) and of chromosome segment substitution line 28 (CSSL-28). The survival rates were determined after a 4-week recovery period. Data are means ± SD (two-tailed Student’s t -test; n = 3 biological replicates). Scale bars = 6 cm. b Location of qCS11-jap on chromosome 11 revealing by LOD score plots. c Fine mapping of the qCS11-jap locus. Left, high resolution mapping. STS11-5, STS11-11, MK21.21, MK21.32, MK21.9, MK22.3, STS11-12 and STS11-13 were molecular markers (Supplementary Data 5 ). Right, survival rates of six recombinants (R1–R6) and the parents. Data are means ± SD (n = 3 biological replicates). d Chilling tolerance of 93-11 and a homozygous recombinant line (R2-7-4). Data are means ± SD (two-tailed Student’s t -test; n = 3 biological replicates). Scale bars = 6 cm. e The expression levels of ORF9 ( LOC_Os11g36200 ) in 93-11 and Nipponbare (NIP) with different treatment times at 4 °C. Data are means ± SD ( n = 3 biological replicates). See also Supplementary Fig. 1 . Source data are provided as a Source Data file. Full size image To clone the major genes underlying qCS11-jap , CSSL-28 was backcrossed with 93-11 then self-crossed to obtain a F 2:3 population. Hundred individuals of the F 2:3 population were used to detect the chilling tolerance and were genotyped using nine markers from the 5.6–23.9 Mb region (Supplementary Data 1 ). LOD score plots revealed that qCS11-jap was within the 2.3-Mb interval between STS11-11 (20.9 Mb) and STS11-12 (23.2 Mb) (Fig. 1b ). All 1800 individuals comprising the F 2:3 population were analyzed, and six recombinants (R1–R6) with recombination between STS11-11 and STS11-12 were selected. The cold tolerance and genotypes of these six recombinants, 93-11 and CSSL-28 were tested to isolate the major gene underlying qCS11-jap . The results showed that the survival rate of R1 without Nipponbare segment in the STS-11-11–MK22.3 region was not significantly different compared with 93-11; the survival rate of R2 with heterozygous segment fell between the rates of 93-11 and CSSL-28. These results indicated that qCS11-jap was located in the region between STS-11-11 and MK22.3. The survival rate of R3 was closer to that of CSSL-28, indicating that qCS11-jap could be further mapped in the region between STS-11-11 and MK21.9. R4–R6 were chilling-sensitive, showing survival rates comparable to that of CSSL-28. The relevant region of qCS11-jap was thus narrowed to the region between MK21.21 and MK21.32 (Fig. 1c ). Sequence analysis showed that there are 9 predicted genes ( ORF1 – ORF9 ) in the 110-kb mapping region (Fig. 1c ). To determine the major gene in this region, a homozygous recombinant line (R2-7-4) was selected from the offspring of the F 2:3 population using molecular markers. R2-7-4 contained the Nipponbare segment from 21.2–22.6 Mb (Supplementary Fig. 1b ). Chilling tolerance test showed that the survival rate of R2-7-4 (15.0%) was significantly lower than that of 93-11 (68.7%) (Fig. 1d ). The expression levels of all 9 predicted genes (Fig. 1c ) within this region in 93-11 and R2-7-4 were detected using transcriptome sequencing after chilling treatment for 0, 4, 24 h. The results showed that the expression of ORF9 was clearly induced by chilling in R2-7-4 (Supplementary Fig. 1c ). To further validate the transcriptome data, the transcript levels of ORF9 in the chilling-treated seedlings of 93-11 and Nipponbare were detected by qRT-PCR. The results showed that ORF9 was consistently induced by chilling in Nipponbare but not expressed in 93-11 (Fig. 1e ). Therefore, ORF9 ( LOC_Os11g36200 ) may be the candidate gene for response to the chilling. COG1 is essential for chilling tolerance in japonica rice To determine whether ORF9 , here designated C hilling-t o lerance in G engdao / japonica rice 1 ( COG1 ) underlies the QTL, two loss-of-function mutants ( cog1-1 and cog1-2 ), mutated by the CRISPR/cas9 approach, and two overexpression lines (OE1 and OE4) were generated in the japonica cultivar Zhonghua 11 (ZH11) (Fig. 2a, b and Supplementary Fig. 2a ). The survival rate of ZH11 was 49% after the chilling treatment for 72 h, while those of cog1-1 and cog1-2 were 15% and 26%, respectively (Fig. 2c ). In contrast, the OE1 and OE2 exhibited higher survival rates (62% and 72%, respectively) than that of ZH11 (9%) when the seedlings were treated for 80 h by cold (Fig. 2d ). In the indica background, on the contrary, both the overexpression lines and the COG1::COG1-HA transgenic lines showed decreased chilling tolerance compared with the wild type 93-11, confirming the chilling-sensitive phenotype of CSSL-28 (Figs. 2e, f and Supplementary Fig. 2b , c ). The genomic sequence analysis data showed that COG1 was disrupted by a 6,665-bp insertion in the indica 93-11 (Supplementary Fig. 2d ), consistent with the qRT-PCR results (Fig. 1e ). This difference between the phenotypes of COG1 -overexpression lines in japonica and indica rice may result from differences in their genetic backgrounds. Such similar case is also seen in other genes [38] , [39] , [40] . Therefore, these results suggest that COG1 positively modulates chilling tolerance in japonica rice, but its invading in indica rice showed a negative regulator. Fig. 2: COG1 is essential for chilling tolerance in japonica rice. a Identification of cog1-1 and cog1-2 via sequencing. PAM, protospacer adjacent motif. b The expression levels of COG1 in ZH11 and two COG1- overexpression lines (OE1 and OE4). Data are means ± SD ( n = 3 biological replicates). c , d The chilling tolerance of COG1 mutants ( cog1-1 and cog1-2 ) ( c ) and COG1- overexpression lines ( d ) in the ZH11 background. The seedlings of mutants and overexpressed lines were treated at 4 °C for 72 h and 80 h, respectively. The survival rates were determined after a 4-week recovery period. Data are shown as the means of three replicates ± SD (two-tailed Student’s t -test). Bar = 6 cm. e The chilling tolerance of COG1::COG1-HA transgenic lines (Line2 and Line4) in the indica 93-11 background. The seedlings were treated at 4 °C for 44 h. Bar = 6 cm. Data are means ± SD (two-tailed Student’s t -test; n = 3 biological replicates). f The chilling tolerance of COG1- overexpression lines (OX1 and OX8) in the 93-11 background. The seedlings were treated at 4 °C for 44 h. Bar = 6 cm. Data are means ± SD (two-tailed Student’s t -test; n = 3 biological replicates). See also Supplementary Fig. 2 . Source data are provided as a Source Data file. Full size image COG1 is selected during japonica rice domestication Sequence comparison between Nipponbare and 93-11 indicated that COG1 of Nipponbare is a 1605-bp open reading frame encoding 534 amino acids, but COG1 of 93-11 contain a 6,665-bp insertion at position +9 from the start codon, resulting in silence of this gene (Fig. 3a and Fig. 1e ). Variation of COG1 sequences were then investigated in natural populations using a pan-genome dataset comprising 67 accessions that represent all major genetic clusters in O. sativa and O. rufipogon [41] , including 23 accessions of O. sativa temperate japonica , 5 of O. sativa tropical japonica , 20 of O. sativa indica , 6 of O. sativa aus and 13 of O. rufipogon (Supplementary Data 2 ). Analysis of the COG1 coding region revealed 12 haplotypes, which could be divided into three groups (haplogroup1 to 3) (Fig. 3a , Supplementary Data 2 and 3 ). All of the selected 28 japonica rice accessions (including Nipponbare) and 3 O. rufipogon varieties (which originated from China) belonged to haplogroup1, which encoded a full-length COG1 protein. In contrast, the haplogroup2 had a 1-bp insertion (T) at position +28 resulting in a frameshift in 9 indica and 3 aus accessions. In addition, the haplogroup3, containing a 6,665-bp insertion at +9, was found in 8 indica (including 93-11) and 2 aus accessions (Fig. 3a , Supplementary Data 3 ). Phylogenetic analysis based on the COG1 sequences of the 67 accessions indicated that clustering among all japonica accessions and the Chinese O. rufipogon accessions carrying the chilling-tolerant haplogroup1 (Fig. 3b and Supplementary Data 3 ). These observations suggested that the haplogroup1 of COG1 originated from Chinese O. rufipogon and was fixed in japonica rice during domestication. Fig. 3: COG1 is selected during japonica rice domestication. a The three COG1 haplogroups identified in 67 representative rice accessions. The Nipponbare genome sequence was used as a reference. b Phylogenetic tree showing the relationships of COG1 haplotypes. Phylogenetic tree was constructed using the sequences of COG1 in 67 representative rice accessions. c Nucleotide polymorphism and neutrality tests for COG1 in the 67 representative rice accessions. S : Number of sample. h : Number of haplotypes. π: Average number of pairwise nucleotide differences per site calculated on the silent sites. D : Tajima’s D value. d The within population selection signal value (SweeD) of the 500-kb region flanking COG1 . See also Supplementary Data 2 and 3 . Full size image To examine whether domestication has acted on COG1 , nucleotide diversity was analyzed in the COG1 sequences of the 67 representative rice accessions. A comparison of the nucleotide diversity among indica , tropical japonica , temperate japonica , aus and O. rufipogon accessions indicated that temperate japonica ( π = 0.00128) exhibited lower diversity than indica ( π = 0.01069), tropical japonica ( π = 0.00292), aus ( π = 0.00486) and O. rufipogon ( π = 0.00589) (Fig. 3c ). Tajima’s D [42] values were calculated for each accession, and significantly negative values were observed only in temperate japonica accessions (Fig. 3c ), indicating that natural selection or genetic bottleneck played a critical role during the northward expansion of rice planting. To further determine this result, SweeD scanning was performed using the resequencing data of the 1176 landraces in the 3000 Rice Genomes Project [8] , [43] , [44] . The result showed that a selection signal was detected only in temperate japonica landraces in the 500-kb region flanking COG1 (Fig. 3d ), suggesting that COG1 had been subject to human artificial selection. Taken together, the COG1 conferring chilling tolerance in japonica rice might represent an ancient allele preserved in Chinese populations of O. rufipogon and selected during domestication of japonica rice. COG1 encodes a plasma membrane and ER localized LRR-RLP COG1 was predicted to encode an LRR-RLP with 17 LRRs based on its DNA sequences (Fig. 4a and Supplementary Fig. 3 ). In order to analyze the subcellular localization, COG1-GFP was expressed in rice protoplasts. The confocal observation showed that fluorescence of COG1-GFP overlapped with that of PIP2-mCherry, a marker for the plasma membrane and endoplasmic reticulum (ER) [45] (Fig. 4b ). To confirm this subcellular localization, the proteins of plasma membrane, ER, cytoplasmic, and nuclear fractions were extracted from the COG1::COG1-HA transgenic rice in the ZH11 background ( COG1-HA -L1) and detected by anti-HA antibody. The immunoblotting results showed that COG1-HA was clearly enriched in the plasma membrane and ER fractions (Fig. 4c ). To analyze the effects of chilling on COG1 accumulation, the seedlings of COG1-HA -L1 were cold-treated then COG1-HA was detected at several timepoints. It was found that relative band densities of COG1-HA were 1.0, 3.2, 6.3, and 12.8 after chilling treatment for 0, 12, 24, 48 h, respectively (Fig. 4d ). Therefore, COG1 encodes a cold-induced LRR-RLP located in the plasma membrane and ER. Fig. 4: COG1 encodes a plasma membrane and ER localized LRR-RLP. a Schematic of COG1 protein structure. Amino acid residues 1 to 53 comprise the signal peptide (SP), and residues 118 to 534 form 17 LRR domains. See also Supplementary Fig. 3a . b Localization of COG1 in rice protoplasts, plasma membrane (upper panel) and ER (down panel). PIP2-mCherry is a marker for the plasma membrane and ER. Scale bar = 10 μm. c Localization of COG1 revealing by immunoblotting assay. The COG1-HA fusion protein in COG1::COG1-HA transgenic rice ( COG1-HA -L1) in the ZH11 background was detected by anti-HA antibody. H + -ATPase, BiP, actin, and histone 3 (H3) were used as markers of the plasma membrane protein (PM), ER protein, cytoplasmic protein (Cyt), and nuclear protein (Nuc), respectively. d COG1 accumulation in COG1-HA -L1 exposed to chilling treatment for 0, 12, 24, and 48 h. The ratio of the intensity of the COG1-HA band to that of the rubisco band at 0 h was set as 1.0. Similar results of b–d were observed from three independent biological repeats. Source data are provided as a Source Data file. Full size image Chilling treatment enhances the interaction between COG1 and OsSERL2 The membrane localized LRR-RLPs can transmit cellular signals through interactions with SERK family members [22] , [23] . Based on the DNA sequences, rice genome is predicted to encode two SERKs and seven SERLs [28] ( http://rice.uga.edu/ ). The interactions between COG1 and these nine OsSERK/OsSERL family members were detected by yeast two-hybrid assays. The data showed that OsSERL2 had a stronger interaction with COG1 than OsSERL4, OsSERL5, OsSERK1 or OsSERK2 did (Supplementary Fig. 4a ). These interactions were further confirmed in plant cells via bimolecular fluorescence complementation (BiFC) assays. COG1-nVenus was co-expressed in rice protoplasts with OsSERL2-cCFP, OsSERL4-cCFP, OsSERL5-cCFP, OsSERK1-cCFP, and OsSERK2-cCFP, respectively. Data showed only the protoplasts co-expressing COG1-nVenus with OsSERL2-cCFP produced a clear YFP fluorescence signal (Supplementary Fig. 4b and Fig. 5a ). Furthermore, co-immunoprecipitation (Co-IP) assays showed that COG1 interacted specifically with OsSERL2 (Fig. 5b ). The confocal observation found that COG1 co-localized with OsSERL2 in the plasma membrane (Supplementary Fig. 4c ). Thus, both in vitro and in vivo data support that COG1 physically interacts with OsSERL2. Fig. 5: Chilling enhances the interaction between COG1 and OsSERL2. a Verification of the interaction between COG1 and OsSERL2 in rice protoplasts using BiFC assay. Empty cCFP and nVenus vectors were used as negative controls. Scale bar = 10 μm. b Co-immunoprecipitation (Co-IP) assay of COG1 and OsSERL2 in rice protoplasts. COG1-HA-GFP and MYC were co-expressed in rice protoplasts as negative controls. “+” or “–”denote the presence or absence, respectively, o f the protein in each sample. c Enhancement of the interaction between COG1 and OsSERL2 by cold in BiFC assay. The numbers at the top of each panels represent fluorescence intensity (mean gray value) as measured by Image J; values were normalized to the fluorescence in protoplasts co-expressing COG1-HA-nVenus and OsSERL2-MYC-cCFP at 28 °C w. Scale bar = 100 μm. d Enhancement of the interaction between COG1 and OsSERL2 by cold in Co-IP assay. The seedlings of COG1-HA -L1/ MYC-OsSERL2 -OE1 (see Methods) were treated at 4 °C for 0, 24, and 48 h and used for Co-IP. The relative intensity of the COG1-HA band was measured by Image J and the lane in COG1-HA -L1/ MYC-OsSERL2 -OE1 at 0 h was set as 1.0. Representative figures of a – d from three biological repeats. See also Supplementary Fig. 4 . Source data are provided as a Source Data file. Full size image To explore the effect of temperature on the interaction between COG1 and OsSERL2, rice protoplasts co-expressing COG1-HA-nVenus and OsSERL2-MYC-cCFP were treated at 28 °C or 4 °C for 24 h, then the fluorescence densities were compared. The confocal observation showed that the fluorescence intensity in protoplasts co-expressing COG1-HA-nVenus and OsSERL2-MYC-cCFP was obviously higher at 4 °C (4.1) than at of 28 °C (1.0), but the protein abundance of COG1-HA-nVenus or OsSERL2-MYC-cCFP was constant after the cold treatment (Fig. 5c and Supplementary Fig. 4d ). To confirm these results, COG1-HA -L1 and COG1-HA -L1/ MYC-OsSERL2 -OE1 seedlings were treated at 4 °C and Co-IP assays were performed with equivalent levels of COG1-HA in the total proteins. The immunoblotting showed that the relative density of COG1-HA band was increased to 4.7 and 5.8 after 24 and 48-hour treatment, respectively, compared with 0-hour treatment (1.0) (Fig. 5d ). Collectively, these results suggested that cold stress strengthen the interaction between COG1 and OsSERL2. COG1 promotes the activation of OsSERL2 for enhancing cold tolerance To understand how COG1 response to cold stress by interacting with OsSERL2, the Tandem Mass Tag (TMT)-labeled high-throughput phosphorylation proteomics approach was used. The mass spectrometry (MS) results showed that the phosphorylation of OsSERL2 at Ser599 was induced after 24-h chilling treatment in ZH11 (Fig. 6a, b and Supplementary Fig. 5a ). To exclude that the induction of phosphorylation of OsSERL2 resulting from the protein accumulation, OsSERL2::OsSERL2-MYC was expressed in rice protoplasts. The protein level of OsSERL2 did not significantly change after the treatment (Supplementary Fig. 5b ). To test the effect of COG1 on cold-induced phosphorylation of OsSERL2, phospho-Ser599 (pSer599) levels of OsSERL2 were detected in ZH11, cog1-1 and COG1 -OE1 using the Parallel Reaction Monitoring (PRM) method [46] . The results showed that pSer599 levels were lower in cog1-1 but higher in COG1 -OE1 than in ZH11 after chilling treatment (Fig. 6c , Supplementary Fig. 5c and Supplementary Data 4 ). The kinase activity of OsSERL2 may have been affected by pSer599, which is in the C-terminal tail of OsSERL2 (Supplementary Fig. 5d ) [47] , [48] . Kinase activity were therefore detected in the cytoplasmic domain of OsSERL2 (OsSERL2-CD, residues 290–641) and a mutated form of OsSERL2-CD, in which Ser599 was substituted with Ala599 (OsSERL2-CD S599A ), using the general substrate myelin basic protein (MBP). The phospho-MBP levels decreased from 1.0 to 0.5 in OsSERL2-CD S599A compared to OsSERL2-CD (Fig. 6d ), implying that the phosphoralation on Ser599 is essential for the activation of OsSERL2. Fig. 6: COG1 promotes the activation of OsSERL2 to enhance cold tolerance. a The volcano plot of TMT-labeled phosphorylation proteomics. Phosphorylation levels are shown for proteins extracted from ZH11 seedlings after treatment at 4 °C for 0 and 24 h. OsSERL2 phosphorylation at Ser599 (pSer599) was induced after 24 h of chilling. Data are shown as the means of three biological replicates (two-tailed Student’s t -test). b The phosphorylation intensity of OsSERL2 at Ser599 identified by TMT-labeled phosphorylation proteomics after treatment at 4 °C for 0, 24 h. Data are shown as the means of three biological replicates (two-tailed Student’s t -test). c Quantification of OsSERL2-pSer599 levels in ZH11, cog1-1 and COG1 -OE1 as identified with LC-MS/MS using the parallel reaction monitoring (PRM) method. The phospho-peptide fragment ions peak area values were normalized by min-max normalization. The detailed data were showed in Supplementary Data 4 . d The influence of pSer599 on activation of OsSERL2 in vitro. Anti-phosphorylated myelin basic protein (pMBP) antibody was used to detect the kinase activity of cytoplasmic domain of OsSERL2 (His-OsSERL2-CD) and a version with a Ser to Ala mutation at site 599 (His-OsSERL2-CD S599A ), and anti-His antibody was used to detect the amount of protein added. “+” or “–”denote the presence or absence, respectively, of the protein in each sample. Similar results were observed from three independent biological repeats. e Kinase activity of MYC-OsSERL2 and MYC-OsSERL2 S599A in ZH11, cog1-1 and COG1 -OE1 seedlings after cold stress. Anti-MYC antibody was used to detect MYC-OsSERL2 and MYC-OsSERL2 S599A in the immunoprecipitation product. Representative figures from three biological repeats. f , g The chilling tolerance of osserl2 mutants ( f ) and MYC - OsSERL2 overexpression lines ( OsSERL2- OE1 and OsSERL2- OE2) ( g ) were treated at 4 °C for 70 h and 84 h. Bar = 6 cm. The survival rates were determined after a 4-week recovery period. Data are means ± SD (two-tailed Student’s t -test; n = 3 biological replicates). h The chilling tolerance of 35 S::MYC-OsSERL2 S599D / cog1-1 ( OsSERL2 S599D / cog1-1 ) and 35 S::MYC-OsSERL2 / cog1-1 ( OsSERL2 / cog1-1 ) seedlings were treated at 4 °C for 78 h. Bar = 6 cm. The survival rates were determined after a 4-week recovery period. Data are means ± SD (two-tailed Student’s t -test; n = 3 biological replicates). See also Supplementary Fig. 5 . Source data are provided as a Source Data file. Full size image Based on the results showing that pSer599 level was affected by COG1 (Fig. 6c ) and appeared essential for kinase activity of OsSERL2 (Fig. 6d ), it can be speculated that COG1 may mediated OsSERL2 kinase activity by regulating pSer599 level. To determine this speculation, the activity of MYC-OsSERL2 was detected in the protoplasts of ZH11, cog1-1 and COG1 -OE1. The immunoblotting results showed that the cold-induced kinase activity of MYC-OsSERL2 was lower in cog1-1 but higher in COG1 -OE1 than in ZH11 after chilling treatment (Fig. 6e ). When Ser599 was mutated to Ala, the kinase activity of MYC-OsSERL2 S599A was weakened in vivo (Fig. 6e ). These results suggested that COG1 promotes the cold-induced activation of OsSERL2 through enhancing pSer599 level. In order to test the function of OsSERL2 in chilling tolerance, loss-of-function mutants ( osserl2-1 and osserl2-2 ) and MYC-OsSERL2 overexpression lines ( OsSERL2- OE1 and OsSERL2- OE2) were generated in the ZH11 background (Supplementary Fig. 5e, f ). After the seedlings were treated at 4 °C for 70 h, the survival rates of osserl2-1 and osserl2-2 (38% and 11%, respectively) were significantly lower than that of ZH11 (63%) (Fig. 6f ). In contrast, the survival rates of the overexpression lines were higher than that of ZH11 after treatment at 4 °C for 84 h (Fig. 6g ). To demonstrate the genetic function of pSer599 in OsSERL2, the 35 S::MYC-OsSERL2 and 35 S::MYC-OsSERL2 S599D (Ser599 was substituted with Asp599 to mimick phospho-Ser) transgenic plants in cog1-1 background were generated. After the seedlings were treated at 4 °C for 78 h, the survival rates of 35 S::MYC-OsSERL2 S599D / cog1-1 (32%) was significantly higher than that of cog1-1 (11%), or that of 35 S::MYC-OsSERL2 / cog1-1 (22%) (Fig. 6h and Supplementary Fig. 5g ). These results suggested that COG1 promotes the activation of OsSERL2 relying on pSer599 to enhance cold tolerance. The COG1-OsSERL2 complex causes the activation of OsMAPK3 to transmit cold signal As known, MAPK cascades are key signaling modules downstream of RLKs/RLPs receptor complexes [29] . OsMAPK3 is a critical protein in the rice MAPK cascade that is specifically induced by chilling [35] , [49] . Our phosphorylation proteomics data also showed that the phosphorylation levels of Thr194 and Tyr196 in OsMAPK3 were induced by chilling (Supplementary Fig. 6a–c ). To confirm whether COG1-OsSERL2 could activate the OsMAPK3 cascade in chilling signaling, the phospho-Thr194 and phospho-Tyr196 levels of OsMAPK3 (pOsMAPK3) were detected in COG1 and OsSERL2 transgenic plants using anti-pTEpY antibody [49] , [50] . Compared with wild-type ZH11, the pOsMAPK3 levels were decreased in cog1-1 (Fig. 7a ) but increased in COG1 overexpression lines after chilling treatment (Fig. 7b ). Furthermore, the pOsMAPK3 levels were also decreased in osserl2-1 but increased in MYC-OsSERL2 overexpression lines compared to ZH11 after chilling treatment (Fig. 7c and d ). Consistent with the antibody assay results, the PRM assay also showed that the pOsMAPK3 levels were decreased in cog1-1 but increased in COG1 -OE1 compared to ZH11 after chilling treatment (Supplementary Fig. 6d, e ). Therefore, the COG1-OsSERL2 complex caused the activation of OsMAPK3 to transmit cold signal from the membrane to the cytoplasm (Fig. 7e ). Fig. 7: The COG1-OsSERL2 complex causes the activation of OsMAPK3 to transmit cold signal. a , b , c and d The phospho-Thr194 and phospho-Tyr196 levels of OsMAPK3 (pOsMAPK3) in cog1-1 ( a ), in COG1 overexpression lines ( COG1 -OE1 and COG1 -OE4) ( b ), in osserl2-1 ( c ), and in MYC - OsSERL2 overexpression lines ( OsSERL2 -OE1 and OE2) ( d ). Total protein extracts were used for immunoblotting with anti-pTEpY and anti-actin antibodies. The relative band intensities were measured with Image J. The ratio of the band intensities of pOsMAPK3 to actin in ZH11 after 4 °C treatment for 0 h was set to 1.0. Representative figures of a–d from three biological repeats. e Working model of COG1. COG1 might originated from Chinese populations of O. rufipogon and been under selection in japonica rice during domestication. The receptor like protein COG1 interacts with OsSERL2 and this interaction is enhanced by chilling. The interaction promotes activation to OsSERL2 for sensing cold signals. The COG1-OsSERL2 complex causes the activation of OsMAPK3 to transmit cold signal from the membrane to the cytoplasm, enhancing cold tolerance in rice. See also Supplementary Fig. 6 . Source data are provided as a Source Data file. Full size image The trait of chilling tolerance is genetically controlled by multiple genetic loci. As known, the chilling tolerance gene COLD1 , which is found in japonica accessions with a specific SNP2, originated from the Chinese population of O. rufipogon [2] . Alternatively, phylogenetic and population genetic analyses here suggested that COG1 in japonica accessions with haplogroup1 originated from Chinese O. rufipogon populations and was fixed in japonica due to strong human selection during domestication (Fig. 3 ). COG1 is a novel major gene of qCS11-jap , which confers chilling tolerance in japonica rice but make sensitive to the tolerance in indica background (Fig. 1 and Fig. 2 ). Natural populations showed that the functional COG1 was fixed only in chilling-tolerant subspecies ( japonica rice) and negatively selected in indica rice (Supplementary Data 3 and Fig. 3 ). Our findings are consistent with archeological and genetic evidence of japonica domestication, japonica rice originated in the Yangtze Valley of China ~9000 years ago then underwent a low-temperature bottleneck, forming both temperate and tropical japonica varieties during a global cooling event ~4200 years ago [7] , [44] . Importantly, our work provides another piece of evidence that temperature is a major factor influencing rice domestication [2] , [3] , [44] . The fixation and extension of favored alleles that enhance chilling tolerance to maintain growth of japonica rice in regions with relatively low yearly temperatures. It is extensive application potential in rice breeding that the epistasis traits of QTL genes depend on the various genetic background [38] , [39] , [40] , [51] , such as COG1 . The opposite phenotype of COG1 transgenic rice in japonica and indica background may be explained with a model of genetic incompatibilities: invasion of COG1 disturbs endogenous OsSERL2 indica function, causing MAPK cascade down-regulation in indica background (Fig. 1 , Fig. 2 and Supplementary Fig. 7 ) [34] , [52] , [53] , [54] , [55] . Specifically, OsSERL2 indica may have evolved a parallel activation pathway aided by intrinsic RLP/RLK in the absence of COG1 ; in indica genome, OsSERL2 has variations to encode the extracellular domain and C-terminal in genome ( https://snp-seek.irri.org/ ). Interaction of exogenous COG1 with OsSERL2 indica may disturb the critical interaction between OsSERL2 indica and intrinsic RLP/RLK, decreasing OsMAPK3 activation (Supplementary Fig. 7 ) [54] , [55] . Thus, exogenous COG1 from japonica rice would disrupt the intrinsic OsSERL2 indica -mediated chilling tolerance signaling pathway in indica background. The epistasis effect between COG1 and a hypothetical factor in indica varieties may therefore inhibit improvement of traits such as cold tolerance. The identified negative effects can be improved with new technology, such as the gene-editing, to break the linkage drag in molecular breeding. This would promote maintenance of cold-tolerance or other key traits in breeding populations when introgression genes between japonica and indica varieties are used in rice production [51] , [56] . It is the first reported that an LRR-RLP (COG1) with a co-receptor (OsSERL2) senses cold for the tolerance. Evidence from the membrane localization, protein interaction and kinase activity dependent on cold stimulating (Figs. 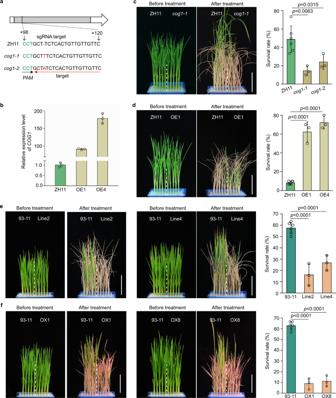Fig. 2:COG1is essential for chilling tolerance injaponicarice. aIdentification ofcog1-1andcog1-2via sequencing. PAM, protospacer adjacent motif.bThe expression levels ofCOG1in ZH11 and twoCOG1-overexpression lines (OE1 and OE4). Data are means ± SD (n= 3 biological replicates).c,dThe chilling tolerance ofCOG1mutants (cog1-1andcog1-2) (c) andCOG1-overexpression lines (d) in the ZH11 background. The seedlings of mutants and overexpressed lines were treated at 4 °C for 72 h and 80 h, respectively. The survival rates were determined after a 4-week recovery period. Data are shown as the means of three replicates ± SD (two-tailed Student’st-test). Bar = 6 cm.eThe chilling tolerance ofCOG1::COG1-HAtransgenic lines (Line2 and Line4) in theindica93-11 background. The seedlings were treated at 4 °C for 44 h. Bar = 6 cm. Data are means ± SD (two-tailed Student’st-test;n= 3 biological replicates).fThe chilling tolerance ofCOG1-overexpression lines (OX1 and OX8) in the 93-11 background. The seedlings were treated at 4 °C for 44 h. Bar = 6 cm. Data are means ± SD (two-tailed Student’st-test;n= 3 biological replicates). See also Supplementary Fig.2. Source data are provided as a Source Data file. 4 – 6 ), as well, downstream responses may suggest the COG1-OsSERL2 complex senses cold to transmit the signaling for tolerance (Fig. 7 ). RLPs typically depend on co-receptor kinases to perceive and respond to cold stress‐induced ligands for activating intracellular signaling; this is analogous to hetero‐dimerization of RLKs [12] , [13] , [22] , [23] . However, no ligand for perceiving the cold signal has been reported in plant cells. 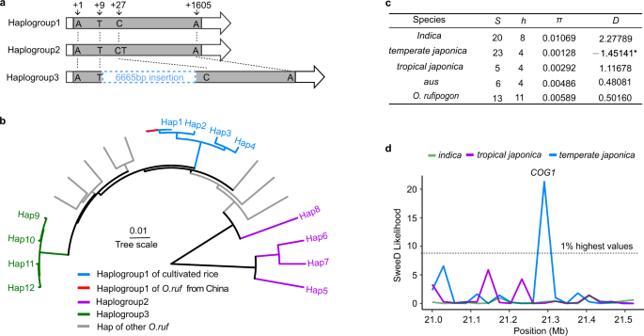Fig. 3:COG1is selected duringjaponicarice domestication. aThe threeCOG1haplogroups identified in 67 representative rice accessions. The Nipponbare genome sequence was used as a reference.bPhylogenetic tree showing the relationships ofCOG1haplotypes. Phylogenetic tree was constructed using the sequences ofCOG1in 67 representative rice accessions.cNucleotide polymorphism and neutrality tests forCOG1in the 67 representative rice accessions.S: Number of sample.h: Number of haplotypes. π: Average number of pairwise nucleotide differences per site calculated on the silent sites.D: Tajima’sDvalue.dThe within population selection signal value (SweeD) of the 500-kb region flankingCOG1. See also Supplementary Data2and3. Changes in the conformation of proteins such as OsCRT3/OsCIPK7 are considered to be another potential mechanism for cold perception in plants [57] , [58] , [59] . The membrane-localized COG1-OsSERL2 complex senses cold through conformational changes, activating the kinase to transduce a signal to the MAPK cascade, ultimately inducing a cold-tolerance response. Conformational changes of the complex to reinforce heterodimerization may be involved in the dynamic cold-sensing process; this could be confirmed in the further through several new approaches, such as, Fourier-transform infrared (FTIR) spectroscopy, Cryo-EM assay [59] , [60] . As known, the sensing of signals in the apoplast by RLK-RLK complexes typically leads to phosphorylation and activation of intracellular domain by transphosphorylation [23] , [29] . With respect to the RLP modulation of RLK in signal sensing, our evidence showed that COG1 may act as an adapter based on its biochemical characteristics (Fig. 4 and Fig. 5 ). Adapter proteins can affect the phosphorylation status of interacting proteins [61] , [62] . Our findings indicate that COG1 affect phosphorylation levels of OsSERL2 at Ser599, regulating kinase activity of OsSERL2 in cold signal transduction (Fig. 6 ). This study uncovered a potential role of the COG1-OsSERL2 complex in perceiving and transmitting the cold signal in rice. Signals including cold, sensed by the RLP-RLK receptor complexes in the membrane are transduced through the MAPK cascade to the cytoplasm (Fig. 7 ) [29] . For example, a cascade involving YDA-MKK4/MKK5-MPK3/MPK6 participates in transmitting stomatal development signal sensed by the AtRLP17-AtSERK3 receptor complex [12] . The OsRLCK185-OsMAPKKKε-OsMKK4-OsMAPK3 cascade transmits chitin-related signal after it is sensed by the OsCEBiP-OsCERK1 complex [63] . The activated OsMAPK3 directly phosphorylates the transcription factors OsbHLH002 [35] or OsWRKY53 [64] , altering the expression of cold-regulated genes. Our phosphoproteomics date also showed an increase of phospho-OsWRKY53 (Supplementary Data 6 ). Here, our data suggest that the activation of OsMAPK3 relied on the COG1-OsSERL2 complex in cold signaling pathway (Fig. 7 ). Overall, our results shed light on a panorama of how a major QTL gene COG1 modulates chilling tolerance in rice. In summary, COG1 is a major gene of the QTL to positively modulate chilling tolerance in japonica rice. COG1 originated from Chinese populations of O. rufipogon and was selected during japonica rice domestication. The LRR-RLP protein COG1 forms a complex with OsSERL2 to promote its activation for sensing cold signal. The COG1-OsSERL2 complex senses and transmits cold signal from the apoplast to the cytoplasm to activate the MAPK cascade, triggering defenses against chilling stress in japonica rice (Fig. 7e ). This novel cold-sensing module is potentially used in molecular design for rice breeding to improve the traits. Genetic population and plant materials The chromosome segment substitution line (CSSL) population was generated by crossing and back-crossing using the chilling-sensitive indica variety 93-11 as the recurrent parent and the chilling-tolerant japonica variety Nipponbare as the donor parent [37] . The chilling-sensitive line CSSL-28 was selected after evaluating the chilling tolerance of CSSLs at seedling stage. For QTL genetic assay, the F 2:3 population consisting 1800 individuals was generated by crossing the CSSL-28 with 93-11, self-crossing the progeny. A homozygous recombinant line (R2-7-4) was obtained from F 2:3 the population through molecular marker assisted selection. The primers used are shown in Supplementary Data 5 . To generate the mutants of COG1 and OsSERL2 through CRISPR/Cas9 genome editing system, the target site sequences 5'-GAACAACAACAGTGAGAAGC-3' ( COG1 ) and 5'-GCTCCCCGGATTTCCTCGT-3' ( OsSERL2 ) were separately cloned into a CRISPR/Cas9 vector linearized with BsaI (Biogle Cat# BGK03) following manufacturer’s instruction. The full coding sequences of COG1 was amplified from cDNA of ZH11 using the primers pUN1301 -COG1 -F/R, then cloned into pUN1301, a binary vector that carries the maize ubiquitin gene promoter; the vector had been linearized with Bam HI and Kpn I (Supplementary Data 5 ). The construct was transformed in ZH11 and 93-11, respectively, to generate COG1 overexpression lines in both backgrounds. The full coding sequences of OsSERL2 was amplified from cDNA of ZH11 using the primers pUN1301- MYC-OsSERL2 -F2/R2 and 6× MYC fragment was amplified from pBI221-OsbHLH002-MYC construct [49] using the primers pUN1301- MYC-OsSERL2 -F1/R1. The two fragments were assembed into pUN1301 (which had been linearized with Bam HI and Kpn I) to generate the pUN1301- MYC-OsSERL2 construct (Supplementary Data 5 ). The construct was transformed in ZH11 to generate MYC - OsSERL2 overexpression line. Genomic DNA of COG1 comprising promoter fragment (1751-bp) and full coding sequences were amplified from ZH11 using the primers COG1::COG1 -F/R. The product was cloned into the pTFLGHAU vector, which had been linearized with ECoRI and BamHI , to obtain the COG1::COG1-HA construct (Supplementary Data 5 ). The construct was transformed in ZH11 and 93-11, respectively, to generate COG1::COG1-HA transgenic lines in both background. Agrobacterium tumefaciens strain EHA105-mediated transformation was used to introduce the constructs into rice [2] . COG1-HA -L1/ MYC-OsSERL2 -OE1 line was obtained by crossing COG1::COG1-HA transgenic line 1 ( COG1-HA -L1 in the ZH11 background) with the MYC - OsSERL2 overexpression line ( MYC-OsSERL2 -OE1). MYC-OsSERL2 and its mutated form with 1795T > G, 1796C > A (Ser599 were mutated to Asp599, MYC-OsSERL2 S599D ) were each amplified from the pUN1301- MYC-OsSERL2 construct (Supplementary Data 5 ). The two products were separately cloned into WMV049 (wimibio), which had been linearied with Kpn I and Bam HI. The resulting constructs were transformed in the cog1-1 background to generate the 35 S::MYC-OsSERL2/cog1-1 and 35 S::MYC-OsSERL2 S599D /cog1-1 transgenic lines, respectively. Chilling treatment Chilling treatments were performed as described in our previous report with slight modifications [65] . The undehulled seeds were surface-sterilized with 0.6% sodium hypochlorite solution for 15 min, then rinsed three times with sterile distilled water. Sterilized rice seeds were immersed in water for 2 days at 30 °C. After germination, seeds were sown in an incubator with Kimura B nutrient solution and the incubators were placed in a greenhouse with a light intensity of 120 μmol·m –2 ·s –1 at 28/25 °C (day/night) cycles and a short-day photoperiod (10-h day/14-h night). After 2 weeks, seedlings were moved to a water bath, and ~3 cm of the aerial tissue was immersed in water for chilling treatment. The water bath was maintained at 3.8–4.1 °C and in a room at 20 ± 2 °C with the same photoperiod as that in the greenhouse. Each replicate contained >24 seedlings with consistent growth. After cold treatment, seedlings were returned to the greenhouse for recovery. The survival rate (percentage of living seedlings out of all tested plants) was determined after a 4-week recovery period. Each treatment was performed independently at least three times. Significan differences between treatment groups were assessed with Student’s t -test. Variations identification, genetic diversity, and phylogenetic analysis The pan-genome dataset (containing 67 representative rice accessions) was downloaded from RicePanGenome website ( http://db.ncgr.ac.cn/RicePanGenome/ ) [41] . Variations in the coding region of COG1 were called using genomes from the entire dataset. COG1 sequences from all 67 representative rice accessions were aligned to construct a phylogenetic tree using the neighbor-joining method in MEGA 5.0 [66] . Nucleotide diversity analyses of COG1 were performed for each rice subspecies group using DnaSP 5.1 [67] . Resequencing data from 3000 Rice Genomes project were downloaded from the Rice SNP-Seek Database ( https://snp-seek.irri.org/ ) [68] . The resequencing data of the 1176 landraces in 3000 Rice Genomes Project were selected as in previous studies [8] , [44] . The likelihood-based selective sweep detection was calculated by ‘SweeD’ with a 1 kb grid size [69] . Protein extraction and immunoblotting Total proteins were extracted from 14-day-old rice seedlings and rice protoplasts using a buffer consisting of 50 mM Tris-HCl (pH 7.5), 150 mM NaCl, 10% glycerol, 5 mM dithiothreitol (DTT), 1% (v/v) protease inhibitor cocktail (P9599, Sigma), 1% (v/v) IGEPAL CA-630, 1 mM phenylmethanesulfonyl fluoride PMSF (PMSF), 1 mM Na 2 MoO 4 ·2H 2 O, 1 mM NaF, 1.5 mM Na 3 VO 4 , and 1% (v/v) protein phosphatase inhibitor cocktails 2 and 3 (Sigma, Cat# P5726 and P0044). For immunoblotting, the proteins were separated by SDS-PAGE (Genscript, Cat# M00661) in 1× MOPS buffer (Genscript, Cat# M00138), then transferred to a PVDF membrane (Millipore Cat# IPVH00010) via electro-transfer at 120 mA for 90 min. The membrane was incubated in blocking buffer (5% w/v nonfat dry milk, 1×TBS, and 0.1% Tween® 20) for 3 h at room temperature, incubated first with the primary antibody for 8 h, followed by the secondary antibody for 1 h (anti-rabbit IgG, Cat# 7074, anti-mouse IgG, Cat# 7076, Cell Signaling Technology, dilution, 1:5000). To analyze the effects of chilling on COG1 accumulation, 14-day-old seedlings of COG1-HA -L1 were treated at 4 °C for 0, 12, 24, and 48 h. The total proteins were extracted for immunoblotting using anti-HA antibody (Sigma, Cat# H6908, dilution, 1:10,000). The same method was used to detect the COG1-HA with anti-HA antibody, MYC-OsSERL2 with anti-MYC antibody (CWBIO, Cat# CW0299M, dilution, 1:3000) and Rubisco with anti- Rubisco antibody (Agrisera, Cat# AS10700, dilution, 1:5000) from the corresponding transgenic rice, respectively. To analyze subcellular localization of COG1, proteins were extracted from cell fractions of COG1-HA -L1 14-day-old rice seedlings using the Minute™ Plasma Membrane Protein Isolation and Cell Fractionation Kit (invent, Cat# SM-005-P). The proteins were detected by SDS-PAGE using anti-HA, anti-H + -ATPase (Agrisera, Cat# AS07260, dilution, 1:5000), anti-BiP (YOUKE, Cat# YKZP054, dilution, 1:2000), anti-actin (Huaxingbio, Cat# HX1843, dilution, 1:5000), and anti-histone 3 (Earthox Cat# E022020, dilution, 1:10,000) antibodies, respectively. Yeast two-hybrid (Y2H) assays Full-length coding sequences of rice SERK/SERL family members and COG1 were amplified from cDNA of ZH11 using the primers shown in Supplementary Data 5 . Amplicons were cloned into the DUALmembrane system vectors pBT3-STE and pPR3-N (Dualsystems Biotech, Cat# P01201-P01229) after the vectors were linearized with Sfi I, respectively. The pBT3-STE -OsSERK/SERLs and pPR3-N -COG1 vectors were transformed into yeast strains NMY51, following the manufacturer’s instructions of DUALmembrane starter kits. Co-IP analysis To verify the interaction between COG1 and OsSERL2 in vivo, the coding sequences of COG1 and a 3× HA fragment were amplified from COG1::COG1-HA construct using the primers pBI221- COG1-HA-GFP -F1/R1 and pBI221- COG1-HA-GFP -F2/R2, respectively. These fragments were assembed into the pBI221 vector, which had been linearized with Xho I and Kpn I (Supplementary Data 5 ). The coding sequences of OsSERL2 and a 6× MYC fragment were amplified from pUN1301- MYC-OsSERL2 construct using the primers pBI221- OsSERL2-MYC -F1/R1 and pBI221- OsSERL2-MYC -F2/R2, respectively. These fragments were inserted into the pBI221 vector after the sequence encoding the GFP-tag was removed with KpnI and SacI (Supplementary Data 5 ). The resulting plasmids were then transfected into rice protoplasts to perform Co-IP (co-immunoprecipitation) assays as previously described [49] . The Co-IP products were immunoprecipitated from the total protein mixtures using Anti-c-Myc Magnetic Beads (Pierce, Cat# 88843), then separated via 8% SDS–PAGE and detected with anti-MYC and anti-HA antibodies. To determine whether cold affected the interaction between COG1 and OsSERL2, the seedlings of COG1-HA -L1/ MYC-OsSERL2- OE1 were treated at 4 °C for 0, 24, and 48 h and the COG1-HA -L1 were treated at 4 °C for 0 h. Total proteins were extracted from the seedlings and adjusted to contain equivalent levels of COG1-HA prior to immunoprecipitation assays. 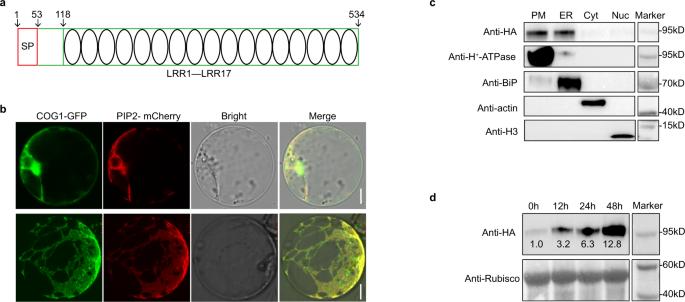Fig. 4:COG1encodes a plasma membrane and ER localized LRR-RLP. aSchematic of COG1 protein structure. Amino acid residues 1 to 53 comprise the signal peptide (SP), and residues 118 to 534 form 17 LRR domains. See also Supplementary Fig.3a.bLocalization of COG1 in rice protoplasts, plasma membrane (upper panel) and ER (down panel). PIP2-mCherry is a marker for the plasma membrane and ER. Scale bar = 10 μm.cLocalization of COG1 revealing by immunoblotting assay. The COG1-HA fusion protein inCOG1::COG1-HAtransgenic rice (COG1-HA-L1) in the ZH11 background was detected by anti-HA antibody. H+-ATPase, BiP, actin, and histone 3 (H3) were used as markers of the plasma membrane protein (PM), ER protein, cytoplasmic protein (Cyt), and nuclear protein (Nuc), respectively.dCOG1 accumulation inCOG1-HA-L1 exposed to chilling treatment for 0, 12, 24, and 48 h. The ratio of the intensity of the COG1-HA band to that of the rubisco band at 0 h was set as 1.0. Similar results of b–d were observed from three independent biological repeats. Source data are provided as a Source Data file. Subcellular localization and BiFC assays To analyze subcellular localization of COG1 in rice protoplasts, the coding sequences of COG1 amplified from cDNA of ZH11 using the primers pBI221 -COG1- F/R, then cloned into pBI221 (which had been linearized with Xho I and Kpn I). To determine whether COG1 co-localized with OsSERL2 in rice protoplasts, the coding sequences of COG1 was amplified using the primers pBI221 -COG1-mCherry- F1/R1 and the mCherry fragment was amplified from the PIP2-mCherry construct [2] using the primers pBI221 -COG1-mCherry- F2/R2. The two fragments were then assembed in the pBI221 vector Kpn I and Sac I. The coding sequences of OsSERL2 was amplified from cDNA of ZH11 using the primers pBI221-OsSERL2-GFP-F/R, then cloned into pBI221 (which had been linearized with XhoI and KpnI ) (Supplementary Data 5 ). For BiFC assays in rice protoplasts, the coding sequences of COG1 , COG1-HA , OsSERL2 , and OsSERL2-MYC were amplified from the pBI221- COG1-HA-GFP and pBI221- OsSERL2-MYC constructions using the primers shown in Supplementary Data 5 , then separately inserted into the pSAT1-cCFP-C and pSAT1-nVenus-C vectors (which had been linearized with Hin dIII and Xba I). The coding sequences of OsSERL4 , OsSERL5 , OsSERK1 , OsSERK2 were amplified from cDNA of ZH11, then cloned into pSAT1-nVenus-C using the same method (Supplementary Data 5 ). Protoplasts were transfected as described above. The transfected protoplasts were observed using a fluorescence microscope (Leica TCS SP5). Images were analyzed with Image LAS-AF software. In vivo phosphorylation assays The phospho-OsMAPK3 levels in Zhonghua 11 (ZH11), cog1-1 , COG1 overexpression lines, osserl2-1 and MYC-OsSERL2 overexpression lines were detected by anti-pTEpY antibody using the method as described in our previous report [49] . In vitro and in vivo protein kinase activity detection For in vitro protein kinase activity detection, the coding sequences of OsSERL2 containing 870–1923 (cytoplasmic domain, OsSERL2-CD) and its mutated form containing a 1795T > G mutation (Ser599 were mutated to Ala599, OsSERL2-CD S599A ) were amplified from the pUN1301- MYC-OsSERL2 construct, respectively. Each amplicon was separately cloned into pColdTF vector which contained a His tag after linearization with Sac I and Xba I (Supplementary Data 5 ). His-OsSERL2-CD and His-OsSERL2-CD S599A were purified by a prokaryotic expression system. A kinase assay was performed in the presence of 50 mM ATP and 30 μL of kinase buffer (25 mM Tris-HCl pH 7.5, 5 mM beta-glycerophosphate, 2 mM dithiothreitol, 0.1 mM Na 3 VO 4 , and 10 mM MgCl 2 .) containing the substrate Myelin Basic Protein (MBP) and either purified His-OsSERL2-CD or His-OsSERL2-CD S599A . Then the mixtures were incubated at 30 °C for 30 min. The reactions were stopped by adding SDS-loading buffer. The reaction mixtures were separated by 12% SDS-PAGE for immunoblotting analysis using anti-His (Earthox, Cat# E022020, dilution, 1:5000) and anti-pMBP (Sigma, Cat# 05-429, dilution, 1:5000) antibodies. For in vivo protein kinase activity detection, the coding sequences of MYC-OsSERL2 and its mutated form containing a 1795T > G mutation ( MYC-OsSERL2 S599A ) were amplified from the pUN1301- MYC-OsSERL2 construct and cloned into pBI221 with Kpn I and Sac I (Supplementary Data 5 ). The resulting plasmids were transfected into protoplasts of ZH11, cog1-1 and COG1 -OE1. The transformed protoplasts were cultured at room temperature for 16 h then at 28 °C or 4 °C for 24 h. After that, total protein was extracted from the protoplasts and immunoprecipitated by Anti-c-Myc Magnetic Beads. The IP products were used for kinase activity detection and performed as described above. Quantitative RT-PCR RNA was extracted from whole seedlings using a plant RNA kit (ZOMANBIO, Cat# ZP405K) following the manufacturer’s instructions. First-strand complementary DNA was synthesized from 2 µg total RNA using a cDNA synthesis kit (YEASEN, Cat# 10911). Quantitative real-time PCR assays were performed using the SYBR Green Realtime PCR Master Mix (TOYOBO, Cat# QPK-201). All primers used for qRT-PCR are given in Supplementary Data 5 . Quantitative phosphoproteomics detection TMT-labeled quantitative phosphorylation detection The 14-day-old rice seedlings of ZH11 were treated at 4 °C for 0, 24 h, then proteins were extracted following previously described [70] . The protein concentration was determined by a BCA kit (Beyotime). Proteins were digested using trypsin (Promega) following the manufacturer’s instruction. For TMT labeling, trypsin-hydrolyzed peptides were desalted with strata XC18 (phenomenex) and freeze-dried under a vacuum. The peptides were dissolved in 0.5 M TEAB and labeled following the manufacturer’s instructions of the TMT-6plex kit (Thermo Fisher, Cat#90068). Phosphopeptide enrichment was performed using a TiO 2 affinity technique (PTM BIO) following the manufacturer’s instruction. The LC-MS/MS analysis were performed as described in our previous report using EASY-nLC 1000 UPLC system and Q ExactiveTM Plus (Thermo Fisher) [70] . The resulting MS/MS data were processed using the MaxQuant search engine (v.1.6.15.0). Tandem mass spectra were searched against the Oryza_sativa_subsp._japonica _39947_PR_20200603.fasta database concatenated with a reverse decoy database. Trypsin/P was specified as the cleavage enzyme and up to two missing cleavages were allowed. The mass tolerance for precursor ions was 20 ppm in the first search and 4.5 ppm in the main search, and the mass tolerance for fragment ions was 0.02 Da. TMT-6plex quantification was performed. The false discovery rate was adjusted to <1% and the minimum score threshold for peptides was >40. For statistical analysis, the mean intensities at 24 h were divided by the mean intensities at 0 h to obtain the phosphorylation intensity ratios of ZH11-24h vs ZH11-0h. Significant differences were assessed with Student’s t -test. To analyze the effects of chilling on OsSERL2 accumulation, OsSERL2 promoter fragment (1710-bp) and the OsSERL2-MYC fragment were amplified from genomic DNA of ZH11 and the pBI221- OsSERL2-MYC construct, respectively. The two fragments were assembed into the pTYLUC vector after removing the sequence encoding the Luciferase-tag with Sac I and Bam HI, resulting in the OsSERL2::OsSERL2-MYC construct (Supplementary Data 5 ). The constructed plasmid was transfected into ZH11 protoplasts, which were treated as described above. After that, total proteins were extracted from the protoplasts and immunoblotting by Anti-MYC antibody. Parallel reaction monitoring (PRM) quantitative phosphorylation detection For PRM, the standard phosphopeptide: “ASGHSTAAADSLSHpSHR” for OsSERL2 and “SDMMpTEpYVVTR” for OsMAPK3 were synthesized. The synthesized standard phospho-peptides were loaded on by gradient and searched by maxquant. Then the retention time (the time elapsed from the start of the sample injected in chromatographic column until the appearance of the apex of chromategram of that sample), m/z values, N-terminal fragments (b ions) and C-terminal fragments (y ions) spectra of the phosphopeptide in the mass spectrum were obtained. These b, y ion spectra were used as the background database. 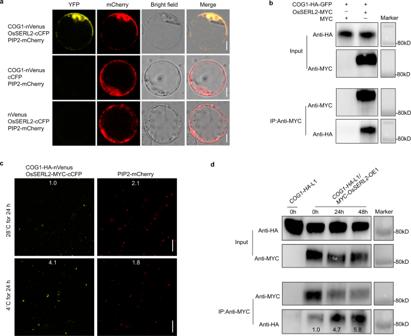Fig. 5: Chilling enhances the interaction between COG1 and OsSERL2. aVerification of the interaction between COG1 and OsSERL2 in rice protoplasts using BiFC assay. Empty cCFP and nVenus vectors were used as negative controls. Scale bar = 10 μm.bCo-immunoprecipitation (Co-IP) assay of COG1 and OsSERL2 in rice protoplasts. COG1-HA-GFP and MYC were co-expressed in rice protoplasts as negative controls. “+” or “–”denote the presence or absence, respectively, o f the protein in each sample.cEnhancement of the interaction between COG1 and OsSERL2 by cold in BiFC assay. The numbers at the top of each panels represent fluorescence intensity (mean gray value) as measured by Image J; values were normalized to the fluorescence in protoplasts co-expressing COG1-HA-nVenus and OsSERL2-MYC-cCFP at 28 °C w. Scale bar = 100 μm.dEnhancement of the interaction between COG1 and OsSERL2 by cold in Co-IP assay. The seedlings ofCOG1-HA-L1/MYC-OsSERL2-OE1 (see Methods) were treated at 4 °C for 0, 24, and 48 h and used for Co-IP. The relative intensity of the COG1-HA band was measured by Image J and the lane inCOG1-HA-L1/MYC-OsSERL2-OE1 at 0 h was set as 1.0. Representative figures ofa–dfrom three biological repeats. See also Supplementary Fig.4. Source data are provided as a Source Data file. 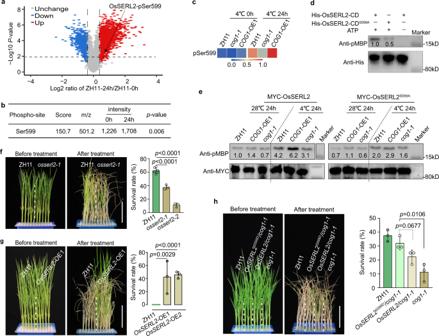Fig. 6: COG1 promotes the activation of OsSERL2 to enhance cold tolerance. aThe volcano plot of TMT-labeled phosphorylation proteomics. Phosphorylation levels are shown for proteins extracted from ZH11 seedlings after treatment at 4 °C for 0 and 24 h. OsSERL2 phosphorylation at Ser599 (pSer599) was induced after 24 h of chilling. Data are shown as the means of three biological replicates (two-tailed Student’st-test).bThe phosphorylation intensity of OsSERL2 at Ser599 identified by TMT-labeled phosphorylation proteomics after treatment at 4 °C for 0, 24 h. Data are shown as the means of three biological replicates (two-tailed Student’st-test).cQuantification of OsSERL2-pSer599 levels in ZH11,cog1-1andCOG1-OE1 as identified with LC-MS/MS using the parallel reaction monitoring (PRM) method. The phospho-peptide fragment ions peak area values were normalized by min-max normalization. The detailed data were showed in Supplementary Data4.dThe influence of pSer599 on activation of OsSERL2 in vitro. Anti-phosphorylated myelin basic protein (pMBP) antibody was used to detect the kinase activity of cytoplasmic domain of OsSERL2 (His-OsSERL2-CD) and a version with a Ser to Ala mutation at site 599 (His-OsSERL2-CDS599A), and anti-His antibody was used to detect the amount of protein added. “+” or “–”denote the presence or absence, respectively, of the protein in each sample. Similar results were observed from three independent biological repeats.eKinase activity of MYC-OsSERL2 and MYC-OsSERL2S599Ain ZH11,cog1-1andCOG1-OE1 seedlings after cold stress. Anti-MYC antibody was used to detect MYC-OsSERL2 and MYC-OsSERL2S599Ain the immunoprecipitation product. Representative figures from three biological repeats.f,gThe chilling tolerance ofosserl2mutants (f) andMYC-OsSERL2overexpression lines (OsSERL2-OE1 andOsSERL2-OE2) (g) were treated at 4 °C for 70 h and 84 h. Bar = 6 cm. The survival rates were determined after a 4-week recovery period. Data are means ± SD (two-tailed Student’st-test;n= 3 biological replicates).hThe chilling tolerance of35S::MYC-OsSERL2S599D/cog1-1(OsSERL2S599D/cog1-1) and35S::MYC-OsSERL2/cog1-1(OsSERL2/cog1-1) seedlings were treated at 4 °C for 78 h. Bar = 6 cm. The survival rates were determined after a 4-week recovery period. Data are means ± SD (two-tailed Student’st-test;n= 3 biological replicates). See also Supplementary Fig.5. Source data are provided as a Source Data file. 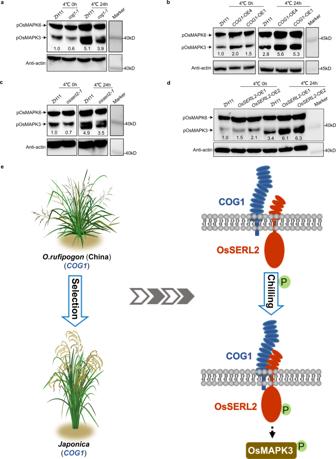Fig. 7: The COG1-OsSERL2 complex causes the activation of OsMAPK3 to transmit cold signal. a,b,canddThe phospho-Thr194 and phospho-Tyr196 levels of OsMAPK3 (pOsMAPK3) incog1-1(a), inCOG1overexpression lines (COG1-OE1 andCOG1-OE4) (b), inosserl2-1(c), and inMYC-OsSERL2overexpression lines (OsSERL2-OE1 and OE2) (d). Total protein extracts were used for immunoblotting with anti-pTEpY and anti-actin antibodies. The relative band intensities were measured with Image J. The ratio of the band intensities of pOsMAPK3 to actin in ZH11 after 4 °C treatment for 0 h was set to 1.0. Representative figures of a–d from three biological repeats.eWorking model of COG1.COG1might originated from Chinese populations ofO. rufipogonand been under selection injaponicarice during domestication. The receptor like protein COG1 interacts with OsSERL2 and this interaction is enhanced by chilling. The interaction promotes activation to OsSERL2 for sensing cold signals. The COG1-OsSERL2 complex causes the activation of OsMAPK3 to transmit cold signal from the membrane to the cytoplasm, enhancing cold tolerance in rice. See also Supplementary Fig.6. Source data are provided as a Source Data file. Total proteins were extracted from 14-day-old rice seedlings of ZH11, cog1-1 and COG1 -OE1 after treatment at 4 °C for 0, 24 h. The protein trypsin digestion and phosphopeptide enrichment were manipulated as described above. The phosphopeptide of each sample was analysed under PRM using the same machine and parameters with LC-MS/MS analysis [46] . Reporting summary Further information on research design is available in the Nature Portfolio Reporting Summary linked to this article.